Broadband electromagnetic cloaking with smart metamaterials The ability to render objects invisible with a cloak that fits all objects and sizes is a long-standing goal for optical devices. Invisibility devices demonstrated so far typically comprise a rigid structure wrapped around an object to which it is fitted. Here we demonstrate smart metamaterial cloaking, wherein the metamaterial device not only transforms electromagnetic fields to make an object invisible, but also acquires its properties automatically from its own elastic deformation. The demonstrated device is a ground-plane microwave cloak composed of an elastic metamaterial with a broad operational band (10–12 GHz) and nearly lossless electromagnetic properties. The metamaterial is uniform, or perfectly periodic, in its undeformed state and acquires the necessary gradient-index profile, mimicking a quasi-conformal transformation, naturally from a boundary load. This easy-to-fabricate hybrid elasto-electromagnetic metamaterial opens the door to implementations of a variety of transformation optics devices based on quasi-conformal maps. On the basis of the invariance of Maxwell’s equations under coordinate transformations, transformation optics (TO) and optical conformal mapping have provided new methods to control electromagnetic fields and wave propagation [1] , [2] . Amongst the celebrated applications of these emerging design approaches is cloaking: making objects of various shapes invisible by implementing coordinate transformations from the physical to a virtual space, in which the concealed object appears to have zero volume [3] , [4] , [5] . The so-called omnidirectional cloaks ‘compress’ an object to a point, rendering it invisible from any direction. The required transformations, however, lead to material requirements that are very difficult to achieve in physical media, such as values of permittivity and/or permeability that are close to zero or very large. Owing to the difficulty of constructing metamaterials with such extreme properties, only a few experimental demonstrations of omnidirectional cloaks exist so far [6] , [7] . On the other hand, the so-called ‘carpet’ or ground-plane cloaks conceptually compress an object to a sheet of infinitesimal thickness. The reduced dimensionality of the compression transformation allows one to select transformations whose implementations require only modest ranges of permittivity, permeability and refractive index [8] . Such devices have been demonstrated to have a large operational bandwidth, the benefit originating from the reduced range of required material properties [9] , [10] , [11] , [12] , [13] , [14] , [15] , [16] . One of the most notoriously difficult properties to achieve without significant dispersion is magnetic permeability. Devices have been proposed for two-dimensional (2D) wave propagation of transverse magnetic waves that use special coordinate transformations combined with eikonal-limit approximations (that is, neglecting the impedance gradient) that allow elimination of the out-of-plane magnetic response, and thus remove the need for any magnetic response [17] . Such approaches are not applicable to transverse electric (TE) wave devices, as TO recipes typically require in-plane magnetic response that cannot be eliminated in the eikonal limit. Fortunately, a special class of transformations exists, known as quasi-conformal maps (QCMs), which minimize or even eliminate deviations of in-plane magnetic permeability from unity. This is achieved by minimizing the degree of anisotropy in the metric tensor of the transformation. A ground-plane cloak is one of the TE-polarization TO devices that can be constructed entirely from dielectric materials as long as a quasi-conformal transformation for a given boundary shape can be found. Because of their ability to realize a much broader range of constitutive properties with considerable control, artificially structured metamaterials have been preferentially used to implement the complex gradient permittivity and permeability distributions required by cloaks and other TO media. In all previously proposed cloaking schemes, the spatial distribution of constitutive parameters is derived assuming interior and exterior cloak boundaries of fixed and known shapes to be hidden. Any deviation in the shape of the hidden object requires a complete redesign of the cloak, and thus a redesign of the metamaterial implementation. In addition, the performance of a TO cloak also degrades with deformations of its exterior boundary, which is exposed to an ambient medium, typically air. Practically unavoidable mechanical loads at the exterior boundary caused, for example, by aerodynamic pressure, can deform conventional metamaterial cloaks beyond the tolerance of their unit cells [18] , [19] . It is therefore important to find recipes for self-compensating, or ‘smart’, TO scenarios. In a smart TO device, the boundary deformation should create a distribution of unit cell deformations that leads to a new distribution of electromagnetic properties that still implements a desired coordinate transformation. That such a behaviour is extremely difficult to achieve in general can be easily understood by considering that the stress and strain distributions of a loaded structure in mechanical equilibrium are solutions of rather complicated equations. Although the strain profiles are uniquely determined by the boundary conditions, obtaining the desired strain distribution throughout the entire volume of the device is very challenging as, in general, this requires knowing the solution to the corresponding inverse problem. An implementation of a given strain profile for a given boundary deformation would require a custom distribution of elastic properties in the entire volume of the device. As difficult as it is to construct such a graded distribution of elastic properties, this resulting distribution of mechanical properties does not solve the smart TO problem; such a distribution would, in general, depend on the type of boundary deformation, meaning, the device would only operate subject to one specific boundary load. Here we propose an elegant practical solution that does not only create the graded-index distribution required for a TO device, but also does it for a virtually arbitrary deformation of the boundary—all with a single ‘smart’ metamaterial. This idea can be quickly grasped from Fig. 1a , where smart ground-plane cloaking is demonstrated in a wide range of deformations of the cloak boundary. This paper provides the first experimental demonstration of a self-adjustable elastic metamaterial for broadband electromagnetic cloaking composed of two triangular regions with a silicone rubber tube array. In the undeformed initial state the tube array is perfectly periodic, with uniform electromagnetic properties homogenized over each unit cell. Both materials involved—silicone rubber and air—are virtually lossless and dispersion-free at microwave frequencies, and the unit cells are electromagnetically non-resonant, which allows broadband operation of the demonstrated device. The uniformity of the array in its initial state and the simplicity of the identical metamaterial elements enable low-cost mass fabrication of large-area devices. Because of its general ability to mimic QCMs, this hybrid elasto-electromagnetic smart metamaterial should have applications in various TO devices not limited to cloaks, as long as they can be implemented with QCMs. 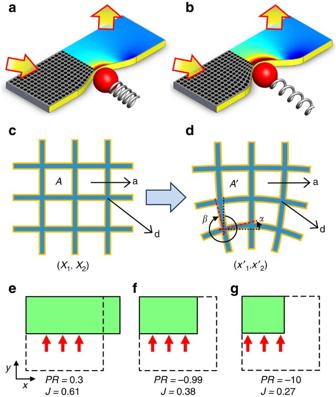Figure 1: Smart cloaking in accordance with the elastic deformation of the cloak boundary. (a,b) Schematics of a smart metamaterial cloaking, which adaptively performs cloaking while we elastically deform the cloak boundary. Arrows indicate the propagation behaviour of incident and reflected beams through cloak, which resembles reflection from a flat reflector. (c,d) The coordinate transformation between the coordinates before (X1,X2) and after (x′1,x′2) the elastic deformation. Frame is incompressible dielectric materials and empty spaces indicate air. Deformation squeezes unit cell air volume (AtoA′) and makes angles of torsion (αandβ). (e–g) Higher negative Poisson’s ratio (PR) minimizes anisotropy of unit cell deformation. When we upwardly compress a square (dashed line) into a half size in y direction, the deformed shape (solid line) and Jacobian (J) are calculated ifPRs are (e) 0.3, (f) −0.99 and (g) −10, respectively. Figure 1: Smart cloaking in accordance with the elastic deformation of the cloak boundary. ( a , b ) Schematics of a smart metamaterial cloaking, which adaptively performs cloaking while we elastically deform the cloak boundary. Arrows indicate the propagation behaviour of incident and reflected beams through cloak, which resembles reflection from a flat reflector. ( c , d ) The coordinate transformation between the coordinates before ( X 1 , X 2 ) and after ( x ′ 1 , x ′ 2 ) the elastic deformation. Frame is incompressible dielectric materials and empty spaces indicate air. Deformation squeezes unit cell air volume ( A to A′ ) and makes angles of torsion ( α and β ). ( e – g ) Higher negative Poisson’s ratio ( PR ) minimizes anisotropy of unit cell deformation. When we upwardly compress a square (dashed line) into a half size in y direction, the deformed shape (solid line) and Jacobian ( J ) are calculated if PR s are ( e ) 0.3, ( f ) −0.99 and ( g ) −10, respectively. Full size image Quasi-conformal transformations with dielectric metamaterials To explain the operation principle of the smart metamaterial cloak, we begin by reviewing general TO theory for TE-polarization devices whose operation is limited to in-plane propagation. An arbitrary 2D coordinate transformation corresponds to an anisotropic transformation of the in-plane tensor of magnetic permeability ( μ ) [1] : where is the Jacobian matrix of the transformation, |G| is its determinant and μ is the permeability tensor in the virtual frame. In the case of cloaks, the relative permeability and permittivity are both unity, μ = ε =1, so that in the virtual space, the cloak mimics electromagnetic properties of free space. The magnetic permeability of a TO cloak is therefore simply μ′ =GG T /|G|. The only situation where a non-trivial (different from identity) transformation does not make μ ′ anisotropic is the case of a conformal transformation. A conformal transformation derives its name from the fact that it conforms to the angle preservation requirement. A conformal transformation thus preserves the sum of the two angles, α and β , of an infinitesimal rectangle (grid element), as shown in Fig. 1c . As any transformation can be seen locally as a combination of a rotation and simultaneous stretching in two orthogonal directions, the conformal requirement thus corresponds to isotropic stretching of a grid element. A conformal transformation therefore has a Jacobian matrix whose two local eigenvalues are equal to each other, so that μ ′=GG T /|G|=1 at each point in the physical space. Thus, by restricting the general coordinate transformations to the subset based on conformal maps, one can come up with implementations of TE-polarization devices not requiring a non-trivial magnetic permeability. On the other hand, the transformation rule for the dielectric constant, ε zz , is very simple: The transformation rule equation (2) holds for any general coordinate transformation, which does not have to be conformal or quasi-conformal. However, if the transformation was not conformal, magnetic permeability would also transform in a non-trivial fashion as equation (1) and become anisotropic. To eliminate the performance limitations arising from the use of non-unity permeability, we thus want to use conformal or close to conformal (quasi-conformal) rather than general coordinate transformations. Design of auxetic smart metamaterials Now, we find a class of electromagnetic metamaterials for TE-polarization problems whose dielectric constant changes as prescribed by the TOs rule of equation (2) as a function of elastic strain. For an elastic deformation, which transforms from ( X 1 , X 2 ) to in Fig. 1c , the deformation gradient tensor ( F ij ) is defined as in solid mechanics and the Jacobian of the deformation gradient tensor ( J =det( F )) is a measure of the volumetric change produced by the elastic deformation, such that d A ′/d A =det( F )= J (ref. 20 ). Smart cloaking requires both sufficient effective permittivity change (Δ ε ) and quasi-conformality in accordance with the deformation of the cloak, whereas μ is unity. The required permittivity change can be realized by use of 2D electromagnetic metamaterials with ε eff = ε ref = ε d f d + ε a f a = ε a +( ε d − ε a ) f d , composed of a dielectric material ( ε d ) and air or free space ( ε a ≈1) with initial volumetric fractions f d and f a (=1− f d ), respectively. Next, we consider what happens to this effective permittivity after an elastic deformation that does not preserve the volume of the metamaterial elements. Such a transformation necessitates the use of compressible materials with Poisson’s Ratio ( PR ) far less than 0.5. If the dielectric material part is incompressible, after an elastic deformation, the volumetric fractions and the effective permittivity of the 2D crystal structure become and , where A ′ is the area of a deformed infinitesimal element with initial area A . The ratio of effective permittivity after and before the deformation is . An elastic and electromagnetic metamaterial makes it possible to perform smart cloaking by this accordingly changing permittivity distribution under the change of the cloak boundary. We observe that in the limit of high dielectric constant of the elastic matrix, that is, ε d >> ε a , the effective permittivity ratio becomes approximately . The effective permittivity varies in proportion to the inverse of the area deformation factor ( A ′/ A ). Note that this equation matches precisely to the TO rule of equation (2), and it does so regardless of the type of transformation used. Now, to ensure ‘smart’ behaviour we need to solve the coupled elastostatics problem, that is, we must ensure that the mechanical equilibrium of a deformed metamaterial grid represents a desired QCM. As described above, this behaviour is needed to maintain a unity permeability in equation (1). One can easily see that an elastic deformation of a homogeneous medium that possesses a negative PR with very large absolute value creates a deformed grid in precise agreement with the conformal transformation requirement. To illustrate this, we compress a square (dashed line) of different PR s of 0.3, −0.99 and −10, choosing a factor of 2 compression in y direction (materials with negative PR are known as auxetics). Elastic deformations (solid line) and Jacobian values ( J ) are calculated using the solid mechanics module of a commercial finite-element software package (COMSOL; Fig. 1e–g ). As we lower the PR , the deformed grid starts to resemble a conformal transformation, and at sufficiently low (negative) values of PR , for instance, −10, it becomes quasi-conformal to high accuracy. Therefore, we can have both ingredients to achieve smart cloaking in a single elasto-electromagnetic metamaterial; the deformed grid closely resembles a quasi-conformal transformation, and the dielectric constant transformation rule matches the one prescribed by TO. To theoretically validate the smart metamaterial cloaking concept, we carried out full-wave electromagnetic finite-element simulations of an incident Gaussian beam, monochromatic with frequency in the microwave X-band (10 GHz) propagating at an angle of 45°. In this work, the smart cloaking behaviour is specifically demonstrated with the reflecting surface of the hidden object parameterized as y = h cos 2 (( x −200)π/125); units in millimetres, with h varying between experiments. 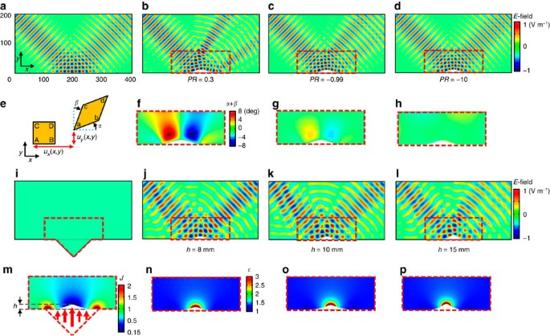Figure 2: Theoretical demonstrations of smart metamaterial cloaking. (a) CalculatedE-field pattern when a Gaussian beam is launched at 45° towards a flat reflecting plane from the left. (b–d) With auxetic smart metamaterial cloak, calculatedE-field patterns when the bottom cloak (red dashed box) boundary is upwardly deformed by 10 mm if (b)PR=0.3, (c)PR=−0.99 or (d)PR=−10. (e) Schematic illustration of the elastic deformation of an infinitesimal element. (f–h) The angle change value,α+β, for the region within the dashed red rectangle inb–dafter the deformation when (f)PR=0.3, (g)PR=−0.99 and (h)PR=−10. (i) Undeformed state of non-auxetic smart cloak within the red dashed polygon. A triangle patch with 125-mm base and 65-mm height is attached to the bottom of the rectangle. (j–l) With non-auxetic smart metamaterial cloak, calculatedE-field patterns when the cloak boundary is upwardly deformed by (j)h=8 mm, (k)h=10 mm and (l)h=15 mm, respectively. (m) Calculated Jacobian values of unit cells (J=det(Fij)) after an elastic deformation for the area in the red dashed line ini. (n–p) Permittivity distributions within the red dashed rectangle inj–lafter deformations with perturbations of (n)h=8 mm, (o)h=10 mm and (p)h=15 mm. Figure 2a shows a simulation of a wave propagating through a material with ε d =50, ε a =1 and f d =0.5, and reflected by a flat reflector. This can be seen as the limiting case of a hidden object of zero height. Then, we increase the height of the object, h , to 10 mm and carry out solid mechanics simulations assuming several different, and progressively lower, PR : 0.3, −0.99 and −10, in Fig. 2b–d , respectively. To test the agreement with conformal requirement, we consider a 2D infinitesimal rectangular material element with dimensions dx × dy , which takes the form of a parallelogram after an elastic deformation ( Fig. 2e ). We calculate the changes of the angle between lines and within the dashed line rectangle after the deformation; Figure 2: Theoretical demonstrations of smart metamaterial cloaking. ( a ) Calculated E -field pattern when a Gaussian beam is launched at 45° towards a flat reflecting plane from the left. ( b – d ) With auxetic smart metamaterial cloak, calculated E -field patterns when the bottom cloak (red dashed box) boundary is upwardly deformed by 10 mm if ( b ) PR =0.3, ( c ) PR =−0.99 or ( d ) PR =−10. ( e ) Schematic illustration of the elastic deformation of an infinitesimal element. ( f – h ) The angle change value, α + β , for the region within the dashed red rectangle in b – d after the deformation when ( f ) PR =0.3, ( g ) PR =−0.99 and ( h ) PR =−10. ( i ) Undeformed state of non-auxetic smart cloak within the red dashed polygon. A triangle patch with 125-mm base and 65-mm height is attached to the bottom of the rectangle. ( j – l ) With non-auxetic smart metamaterial cloak, calculated E -field patterns when the cloak boundary is upwardly deformed by ( j ) h =8 mm, ( k ) h =10 mm and ( l ) h =15 mm, respectively. ( m ) Calculated Jacobian values of unit cells ( J =det( F ij )) after an elastic deformation for the area in the red dashed line in i . ( n – p ) Permittivity distributions within the red dashed rectangle in j – l after deformations with perturbations of ( n ) h =8 mm, ( o ) h =10 mm and ( p ) h =15 mm. Full size image which is supposed to be zero for a precisely conformal mapping ( Fig. 2f–h ) [20] . If we use a typical material with positive PR of 0.3, the mapping condition is not exactly conformal and the bump is not completely hidden. Figure 2b show that a strongly scattered secondary beam is produced and a power gap from the primary scattered beam appears as a result of the bump on the reflector. With PR =−0.99, the angle change α + β is substantially lower; however, the reflected beam still has a noticeable power gap ( Fig. 2c ). When the deformed material is an auxetic material possessing a negative PR with a large absolute value of −10, we observe a nearly conformal map such that the angle change α + β is close to zero ( Fig. 2h ). As a result of a very close match between the transformed permittivity map and the one prescribed by the carpet cloak design, the power gap (an indication of the bump on the reflector) is no longer present ( Fig. 2d ) and the reflected beam is restored as if the wave propagates through a homogenous medium and is reflected by a perfectly flat ground plane. An arbitrary mechanical deformation of a bounded piece of an auxetic material with PR <<−1 is given by a certain conformal transformation. Therefore, auxetic materials provide a smart way to deliver angle-preserving coordinate transformations needed for quasi-conformal TO. The theoretical results shown in Figs 1 – 2 clearly demonstrate that the elastic deformation becomes progressively closer to an exact conformal map as the absolute value of a negative PR increases. Auxetic materials with negative PR between −1 and 0 have been known for a long time [21] , as this range can be implemented in media with all-positive bulk and shear moduli. The regime with PR <−1 requires negative elastic shear modulus; the possibility of auxetic materials with negative PR (0 to −14) and negative shear modulus have been reported recently [22] , [23] , [24] . Design of non-auxetic smart metamaterials In practice, auxetic materials with both highly negative PR and large, positive dielectric constant ( ε d >> ε a ) are not easily realizable. As ε d is not large enough in comparison with ε a in our experimental samples, we introduce an additional structural part at the bottom (a triangular patch) to help achieve the extremely small value of the Jacobian needed for smart cloaking. For example, if ε d =2.88, ε a =1 and f d =0.15, which is close to our experimental conditions, the transformation rule of effective permittivity becomes . For the proper operation of this carpet cloak, the maximum permittivity variation up to (after an elastic deformation) is required, which necessitates J ~0.19. To achieve the desired range of variation for effective permittivity, we attach an additional triangular patch of material with a 125-mm base and 65-mm height to the bottom of the sample ( Fig. 2i ), which gives us deformation Jacobian values as small as 0.19 ( Fig. 2m ). In the experimental demonstration of smart cloaking, we place our elastic metamaterial structure on top of the bump, and create an elastic deformation of the boundary, resulting in curved surfaces of height h =8 mm ( Fig. 2j ) and h =10 mm ( Fig. 2k ), respectively. In both cases of our simulations, the cloaked bumps with different cloak boundaries produce a single specularly reflected beam that would be produced by a perfectly flat ground plane, which implies invisibility of the bump underneath the metamaterial structure. When we further deform the smart cloak with bump height h =15 mm, a strongly scattered secondary beam appears, indicating the deformation limit at which the metamaterial behaves as a carpet cloak ( Fig. 2l ). The effective permittivity distributions within the rectangle in dashed line after deformations of h =8, 10 and 15 mm are shown in Fig. 2n–p , respectively. These results demonstrate that the smart cloak gives the observer the impression of looking at a flat surface for a variety of shapes and heights of the physical bump on the bottom plane. As the bump is covered with a reflector that shields electromagnetic fields from its interior, the volume of its interior can be used as an invisible cavity. Fabrication of smart metamaterials Auxetic materials with very high dielectric constant and negative PR are difficult to realize, and we performed a more feasible experiment using a lower dielectric constant material. In our experiment, a silicone rubber ( ε d ) elastic crystal structure with empty air space ( ε a ) was used, where ε d =2.88 and ε a =1, and the initial volumetric fraction ( f d ) of our sample is f d =0.15 ( Fig. 3a ). The structure is made of a square lattice array of flexible silicone rubber tube with 10 mm outer diameter and 10 mm lattice constant (inset of Fig. 3a ). The empty air space has two regions: the inside tube region with 9 mm inner diameter and interstitial regions between unit rubber tubes. The smart carpet cloak is composed of two triangular regions (marked as C1, C2) made of uniform tube array, serving as a homogeneous medium with an effective index of 1.28 ( Fig. 3a ). The lower triangular region (marked as C1) is elastically compressed to a curved surface with maximum height of h , resulting in a spatially varying density of silicone rubber, embedded in the empty air space ( Fig. 3b ). The spatial distribution of silicone rubber causes a variation of the effective index of refraction across the surface. As we appropriately achieve a smart cloaking device out of a uniform elastic crystal structure, this self-adjustable cloak facilitates easy fabrication in large area and potential applications. By changing the Jacobian ( J ), we are able to span the required effective permittivity range of 1.28–2.88 (inset of Fig. 3b ). 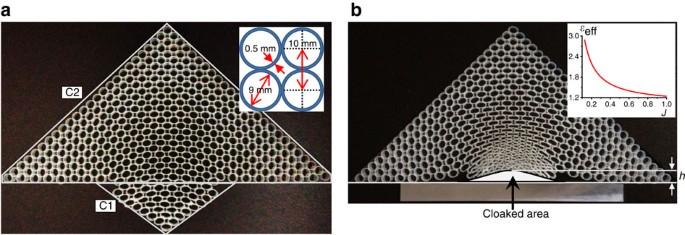Figure 3: Experimental sample of non-auxetic smart metamaterial cloak. Photographs of the sample used in our experiment with an additional triangle patch of 125-mm base and 65-mm height. Images of the sample (a) before and (b) after the deformation. The inset inais a diagram of elastic crystal structure and the inset inbis the effective permittivity curve versus Jacobian values. To prevent refraction at air-sample interface, upper part of cloak has a right-angled triangle shape. Figure 3: Experimental sample of non-auxetic smart metamaterial cloak. Photographs of the sample used in our experiment with an additional triangle patch of 125-mm base and 65-mm height. Images of the sample ( a ) before and ( b ) after the deformation. The inset in a is a diagram of elastic crystal structure and the inset in b is the effective permittivity curve versus Jacobian values. To prevent refraction at air-sample interface, upper part of cloak has a right-angled triangle shape. Full size image The size of the unit cell, 10 mm, is substantially less than the wavelength of microwave radiation at 10 GHz. Therefore, this periodic structure operates in its lowest, ‘acoustic’, branch of the dispersion relation, where it can be generally regarded as an effective medium or ‘metamaterial’ from the electromagnetic properties point of view. We place and reversibly compress the smart metamaterial cloak made of an initially homogeneous medium by pushing it with a triangular bump made of nearly perfect electric conductors. As explained above, the deformation in a specific range always results in some effective permittivity profile that mimics a quasi-conformal coordinate transformation; thanks to the properly chosen elastic properties of the elastic tube array. As in the earlier ground-plane cloak experiments, the purpose of the device is to generate a reflected beam indistinguishable from a specular reflection from a flat, undeformed, conducting surface (‘ground’). Observation of smart metamaterial cloaking effect To verify the predicted behaviour of smart cloaking, the device was tested by launching microwave at 8–14 GHz, incident on the reflecting surface at an angle of 0°–90°, then mapping the TE field distribution inside a planar waveguide. To observe the smartness of the self-adjustable carpet cloak, we place and reversibly compress the smart metamaterial cloak by pushing it with a metallic bump. Then, the measurements of the electric field map profiles at 10 GHz with 45° incident angle were carried out over a wide range of perturbations from h =0 mm to h =11 mm, as plotted in Fig. 4a–h , respectively. For the perturbations below h =2 mm ( Fig. 4a ), the additional patch (C1 in Fig. 3a ) introduces so high refractive index in the centre area, just like a convex lens, that the reflected beam focusing appears [25] . For a broad perturbation range from h =4 mm to h =8 mm ( Fig. 4c–e ), the scattered beam profile shows a singular beam without a power gap, that is, the cloak performance is largely unaffected by the shape of cloak boundary in a specific range. For the perturbations above h =9 mm ( Fig. 4f–h ), the cloak performance suffers, as the effective permittivity change due to the deformation is not sufficient to cover carpet cloaking, causing a strongly scattered secondary beam with a power gap and breakdown of the carpet cloaking. The upward deformation limit for the self-adjustable smart cloak is ultimately restricted by the permittivity magnitude ( ε d ) of the dielectric material. Without a cloak, as shown in Fig. 4i , the presence of a perturbation on the surface ( h =6 mm) produces a strongly scattered secondary beam with a power gap. The reflecting scattered wave interferes with the incident wave and the fringe patterns, shown in the electric field map of Fig. 4 , make it confusing to evaluate the performance of cloaking devices. To remove the interference effects between incident and scattered waves, we average the field map over the region of a wavelength distance to obtain the beam profiles at the reflecting output region as shown in Fig. 5 . 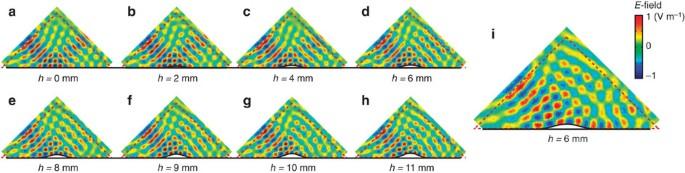Figure 4: Experimentally measuredE-field mapping of the smartly cloaked perturbations and non-cloaked perturbation at 10 GHz. After we place and compress the self-adjustable smart cloak around the perturbation or a ground, a beam incident on the smartly cloaked (a) ground (h=0 mm) and the smartly cloaked bump with perturbations of (b)h=2 mm, (c)h=4 mm, (d)h=6 mm, (e)h=8 mm, (f)h=9 mm, (g)h=10 mm and (h)h=11 mm, respectively. (i) Without the smart cloak, a beam incident on the perturbation ofh=6 mm. The triangle in red dashed line presents the size of sample. Figure 4: Experimentally measured E -field mapping of the smartly cloaked perturbations and non-cloaked perturbation at 10 GHz. After we place and compress the self-adjustable smart cloak around the perturbation or a ground, a beam incident on the smartly cloaked ( a ) ground ( h =0 mm) and the smartly cloaked bump with perturbations of ( b ) h =2 mm, ( c ) h =4 mm, ( d ) h =6 mm, ( e ) h =8 mm, ( f ) h =9 mm, ( g ) h =10 mm and ( h ) h =11 mm, respectively. ( i ) Without the smart cloak, a beam incident on the perturbation of h =6 mm. The triangle in red dashed line presents the size of sample. 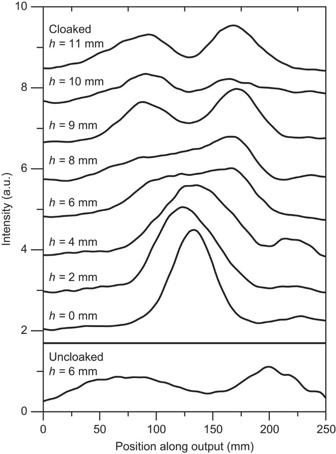Figure 5: Averaged beam profiles of the reflecting scattered waves at the output plane. To remove the interference effects, averaged beam profiles at the output region are presented with a smart metamaterial cloak dependent on the perturbations ofh=0, 2, 4, 6, 8, 9, 10 and 11 mm. Without a cloak, a strongly scattered secondary beam appears. Full size image Figure 5: Averaged beam profiles of the reflecting scattered waves at the output plane. To remove the interference effects, averaged beam profiles at the output region are presented with a smart metamaterial cloak dependent on the perturbations of h =0, 2, 4, 6, 8, 9, 10 and 11 mm. Without a cloak, a strongly scattered secondary beam appears. Full size image To confirm that the cloaking effect persists in a broadband (with instantaneous bandwidth no less than 10%), the device was tested by launching microwave between 8 and 14 GHz, incident on the reflecting surface at an angle of 45°, then mapping the TE field distribution inside a planar waveguide. With a smart metamaterial cloak pushed by a metallic perturbation of height h =6 mm at 45° incidence, the electric field profiles were measured at the frequencies of 8, 11, 12 and 14 GHz, as plotted in Fig. 6a–d , respectively. The dispersion curve of silicone rubber bulk (see Fig. 6e ) shows that the permittivity of silicone rubber is not sensitively changing over the broadband frequency range. Apparently, the device operates fairly well in this experimental setup in the 8–12 GHz range, especially at the 11 and 12 GHz test frequencies. The observation of Gaussian beam cloaking at 8 GHz is complicated by the dimensions of the experimental setup and the diffraction limit for the Gaussian beam waist ( Fig. 6a ). At the other extreme (14 GHz), the metamaterial unit cell is not small enough relative to the wavelength to be accurately homogenizable. This explains the poor performance observed in Fig. 6d . 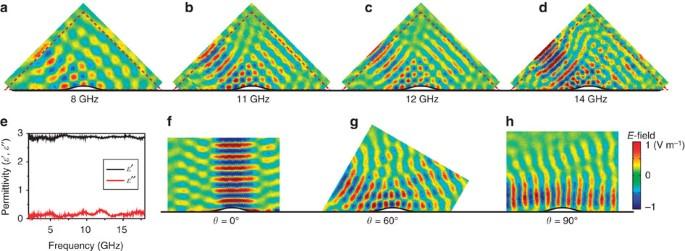Figure 6: Experimentally measuredE-field mapping of smart metamaterial cloaking. MeasuredE-fields depending on frequency and incident angle with a perturbation ofh=6 mm. (a–d) ExperimentalE-field mapping at various frequencies of (a) 8 GHz, (b) 11 GHz, (c) 12 GHz and (d) 14 GHz. (e) Dispersion curve of silicone rubber. (f–h) ExperimentalE-field mapping at various incidence angles of (f) 0°, (g) 60° and (h) 90°. Figure 6: Experimentally measured E -field mapping of smart metamaterial cloaking. Measured E- fields depending on frequency and incident angle with a perturbation of h =6 mm. ( a – d ) Experimental E -field mapping at various frequencies of ( a ) 8 GHz, ( b ) 11 GHz, ( c ) 12 GHz and ( d ) 14 GHz. ( e ) Dispersion curve of silicone rubber. ( f – h ) Experimental E -field mapping at various incidence angles of ( f ) 0°, ( g ) 60° and ( h ) 90°. Full size image An ideal carpet (ground-plane) cloak cancels the reflection spectrum of an object illuminated by plane waves incident from any direction, leaving only the specular reflection of the ground plane itself. To study the incidence angle dependence of our experimental sample, the device, installed in the same parallel plate waveguide, was tested by launching TE-polarized microwave beams at 10 GHz, incident on the reflecting surface at angles from 0° to 90° with respect to the normal. With the smart metamaterial cloak pushed by a metallic object of height h =6 mm, the electric field profiles at 10 GHz were measured at the selected incidence angles of 0°, 60° and 90° with respect to the normal, as plotted in Fig. 6f–h , respectively. These results show that the device operates as a carpet cloak for beams incident at various angles. These results represent an experimental demonstration of a self-adjustable ‘smart’ invisibility cloaking device at microwave frequencies, made of an initially uniform dielectric elastic meta-crystal whose electromagnetic and mechanical properties are homogenizable. The demonstrated smart cloak is nearly lossless and broadband (10–12 GHz), can be extended to covering objects of larger area, and is amenable to inexpensive fabrication. Its ‘smart’ electromagnetic constitutive tensors derive from a combination of electromagnetic and elastic properties. This hybrid elasto-electromagnetic metamaterial approach should have a variety of applications based on quasi-conformal TOs. Derivation of the angle change α + β for conformality test To test the conformality under a coordinate transformation, as described in Fig. 2e , we consider an initial 2D infinitesimal rectangular material element unit cell ( ABCD ) with dx × dy dimensions, which takes the form of a parallelogram ( abcd ) after an elastic deformation. The change of the angle between lines and after the deformation is the same as the sum of angle changes from perpendicular axes, α + β . For a precisely conformal mapping, for example, α =− β and the unit cell preserves the angle after the solid-mechanical deformation. α + β =0 indicates that there is no shear strain ( γ xy = α + β ) in this mechanical deformation. The mechanical deformation of unit cell ABCD into abcd can be represented by displacement . Using the relations of displacements, the shear strain ( γ xy ) is described as When the shear strain is close to zero, the mechanical deformation is also close to conformal mapping condition. Electric field measurements To map the TE field distribution of the scattering region, including the incident and scattered beams, we use a phase-sensitive, near-field microwave scanning system inside a planar waveguide. From a standard X-band coax-to-waveguide coupler, the microwaves are launched into the planar waveguide and the beam is arbitrarily chosen to be incident on the ground plane at an angle of 0°–90° with respect to the normal. The sample was tested with 8–14 GHz wave, then capturing the TE field image on the xy plane. Elastic crystal fabrication For a periodic and uniform elastic crystal, we use injection-moulded silicone rubber tube with 10 mm outer diameter and 9 mm inner diameter. The silicone rubber’s dielectric properties are shown in Fig. 6e . The silicone rubber tube was cut into slices of 10 mm length, then bonded to each other using RTV adhesive. How to cite this article: Shin, D. et al. Broadband electromagnetic cloaking with smart metamaterials. Nat. Commun. 3:1213 doi: 10.1038/ncomms2219 (2012).